Halogen-bonded mesogens direct polymer self-assemblies up to millimetre length scale Aligning polymeric nanostructures up to macroscale in facile ways remains a challenge in materials science and technology. Here we show polymeric self-assemblies where nanoscale organization guides the macroscopic alignment up to millimetre scale. The concept is shown by halogen bonding mesogenic 1-iodoperfluoroalkanes to a star-shaped ethyleneglycol-based polymer, having chloride end-groups. The mesogens segregate and stack parallel into aligned domains. This leads to layers at ~10 nm periodicity. Combination of directionality of halogen bonding, mesogen parallel stacking and minimization of interfacial curvature translates into an overall alignment in bulk and films up to millimetre scale. Upon heating, novel supramolecular halogen-bonded polymeric liquid crystallinity is also shown. As many polymers present sites capable of receiving halogen bonding, we suggest generic potential of this strategy for aligning polymer self-assemblies. Self-assembly of polymers has received significant attention aiming at simple and low-cost methods for new technologies [1] , [2] , [3] , [4] , [5] . Supramolecular principles further allow hierarchical polymeric structures, modularity, complexity and functionalities [6] , [7] , [8] , [9] , [10] . Self-assembly of polymers results in microphase-separated domains at a length scale of ca. 10–100 nm. However, typically the structures are local, that is, they lack common alignment and therefore the materials are macroscopically disordered. To achieve overall alignment in bulk matter, large electric, magnetic and flow fields have been used [11] , [12] , [13] , [14] . In films, graphoepitaxy and surface templating allow long-range order [15] , [16] , [17] , [18] , [19] . Also extensive thermal or solvent annealing [20] classically improve the overall order. However, achieving aligned and globally ordered self-assembled polymer systems organized up to millimetre length scale through simple, rapid and technologically relevant ways remains a fascinating challenge, in order to exploit the properties of the nanometre structures at macroscopic scale. Towards tackling such a problem, we designed self-assemblies involving polymers and low-molecular-weight rod-like mesogens where the latter ones would pack in strictly parallel fashion leading to an overall broken symmetry, where the interface curvature in the local and global scale between the rods and the polymer matrix is minimized, and where plasticization by supramolecular binding of low-molecular-weight units improves dynamics to reach the equilibrium. Such features may synergistically result in an overall spontaneous organization up to macroscale without the need of external stimuli. The aimed strong repulsion of the mesogenic rods from the organic polymeric domains could be achieved by the use of perfluorinated molecules. To this purpose, we used iodoperfluoroalkanes (IPFAs) that can be halogen-bonded to polymers possessing electron-donor sites [21] , [22] , [23] , [24] , [25] . However, in spite of its strength, specificity and directionality, halogen bonding has seldom been used for directing polymer self-assembly [26] , [27] . Here we report, as a model material, the amine hydrochloride derivative of a 4-arm polyethylene glycol, that is, C-[CH 2 -(OCH 2 CH 2 ) 29 -NH 3 + Cl − ] 4 (molecular weight of 5 kDa, a branched semicrystalline polymer, see Methods), halogen-bonded to mesogenic IPFAs ( Fig. 1 ). A star-shaped polymer is selected aiming to reduce coiling and entanglement tendency, which we expect to promote ordering and to allow a dense packing of the noncovalently bonded IPFA chains. In IPFAs, the fluorine atoms inductively boost the electron accepting ability of the terminal iodine, which promotes halogen bonding. The long-chain IPFAs adopt all-trans conformations, showing rod-like behaviour and exceptionally high repulsion from hydrocarbons (fluorophobic effect) [28] . However, selection of proper perfluoroalkyl chain lengths of IPFA turned out to be subtle: too short chains lead to excessive volatility thus reducing the stability of the complexes, whereas too long chains do not allow solution processing to prepare the complexes. Therefore, 1-iodoperfluorodecane (I-C 10 F 21 ) and 1-iodoperfluorododecane (I-C 12 F 25 ) are here selected. Halogen bonds are expected to occur between the chloride anions and the iodine atoms ( Fig. 1 ). The simplicity and rapidity of the method described here demonstrate that the synergistic use of halogen bonding and fluorophobic effect constitutes a major advancement to obtain nanostructured polymeric materials aligned up to the macroscopic scale. 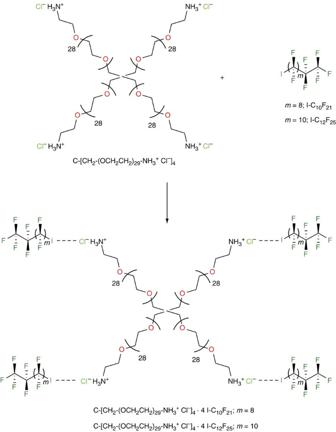Figure 1: Halogen-bonded complex formation. The supramolecular complexes are here denoted as C-[CH2-(OCH2CH2)29-NH3+Cl−]4·4 I-C10F21and C-[CH2-(OCH2CH2)29-NH3+Cl−]4·4 I-C12F25based on their nominal stoichiometric compositions. Figure 1: Halogen-bonded complex formation. The supramolecular complexes are here denoted as C-[CH 2 -(OCH 2 CH 2 ) 29 -NH 3 + Cl − ] 4 ·4 I-C 10 F 21 and C-[CH 2 -(OCH 2 CH 2 ) 29 -NH 3 + Cl − ] 4 ·4 I-C 12 F 25 based on their nominal stoichiometric compositions. Full size image Stoichiometry of the halogen-bonded complexes In small-molecule co-crystals, the chloride anions may behave as either mono- or bi-dentate halogen bond acceptors (see Supplementary Note 1 ). Therefore, to establish the nominal halogen bonding stoichiometry in the present polymeric case, we first used a facile process, where powders of the polymer and I-C 10 F 21 were ground together in a mortar and pestle for 10 min using 1:1 and 1:2 molar ratios of Cl − :I (see Methods). Fourier transform infrared spectroscopy (FTIR) showed that the C-F stretching mode at 1,198 cm −1 and the I-CF 2 deformation mode at 631 cm −1 of I-C 10 F 21 exhibit a blue shift of around 8 and 11 cm −1 upon complexation to the polymer ( Fig. 2a ). Similar blue shift is also observed for the C–O–C bending at 1,100 cm −1 , whereas a smaller blue shift of ca. 2 cm −1 involves the stretching mode of the polymer at 2,880 cm −1 . An intensity decrease in the complex is observed in the region 3,700–3,300 cm −1 , potentially associated with the modified interaction environment of the ammonium chloride group. The spectral changes support supramolecular interaction. Importantly, the 1:1 and 1:2 molar ratios of Cl − :I yielded almost indistinguishable FTIR spectra. Therefore, we suggest that each chloride nominally binds one IPFA molecule, and in the process of grinding the Cl − :I 1:2 composition, the additional IPFA sublimes off the powder owing to its high vapour pressure. Similar FTIR spectra are observed in the complex with I-C 12 F 25 (see Supplementary Fig. 1 ). 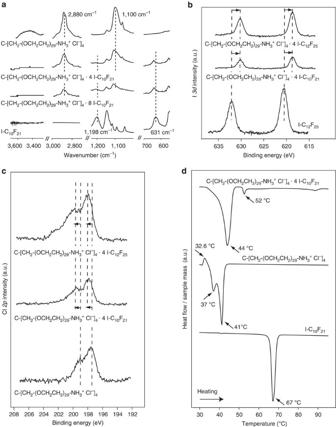Figure 2: Characterization of the halogen-bonded complexes. (a) Attenuated total reflectance (ATR) FTIR spectra in the relevant regions. (b) XPS spectra showing the shifts in I3dand (c) Cl2porbital binding energies upon halogen bonding. (d) DSC thermographs upon the first heating cycle at 10 °C min−1of the starting compounds and the C-[CH2-(OCH2CH2)29-NH3+Cl−]4·4 I-C10F21complex prepared by grinding. Figure 2: Characterization of the halogen-bonded complexes. ( a ) Attenuated total reflectance (ATR) FTIR spectra in the relevant regions. ( b ) XPS spectra showing the shifts in I 3d and ( c ) Cl 2p orbital binding energies upon halogen bonding. ( d ) DSC thermographs upon the first heating cycle at 10 °C min −1 of the starting compounds and the C-[CH 2 -(OCH 2 CH 2 ) 29 -NH 3 + Cl − ] 4 ·4 I-C 10 F 21 complex prepared by grinding. Full size image Further evidence of the halogen bond between C-[CH 2 -(OCH 2 CH 2 ) 29 -NH 3 + Cl − ] 4 and I-C 10 F 21 at the nominal 1:1 Cl − :I molar ratio is given by X-ray photoelectron spectroscopy (XPS) ( Fig. 2b,c ). The complexes were prepared upon mixing the starting materials in isopropanol (see Methods). We expected that upon halogen bonding the electron density of the I atom (halogen bond donor) would increase while that of the Cl − anion (halogen bond acceptor) would decrease, resulting in a downshift of the binding energies for the I 3d doublet of I-C 10 F 21 and an upshift of the Cl 2p doublet in C-[CH 2 -(OCH 2 CH 2 ) 29 -NH 3 + Cl − ] 4 . Measuring the XPS spectrum of highly volatile I-C 10 F 21 posed challenges in our setup under its high-vacuum conditions and focused beam, and therefore the binding energy for the I 3d doublet was measured using the less volatile I-C 12 F 25 . As XPS only probes the nearest atomic neighbourhood of the iodine, the slightly different alkyl tail length is not expected to be relevant in this case. Indeed, the peaks at 620.4 and 632 eV, corresponding to I 3d , shift to 618.7 and 630.2 eV, respectively, while the Cl 2p doublet in C-[CH 2 -(OCH 2 CH 2 ) 29 -NH 3 + Cl − ] 4 shifts to higher energies (see Supplementary Note 2 ). These energy shifts agree with literature values for related interactions [27] , supporting that chloride ion and the IPFA are halogen bonded. Liquid-crystalline behaviour Differential scanning calorimetry (DSC) shows a single sharp endothermic peak at 67 °C for I-C 10 F 21 upon heating ( Fig. 2d ). As polarized optical microscopy (POM) ( Fig. 3b ) shows transition from an optically anisotropic state to an isotropic state upon heating, we assign this as melting. C-[CH 2 -(OCH 2 CH 2 ) 29 -NH 3 + Cl − ] 4 polymer shows the main melting at 41 °C as well as a small exothermic peak at around 33 °C ( Fig. 2d ) due to cold crystallization and related melting endotherm at 37 °C, signalling polymorphism. The corresponding POM images ( Fig. 3a ) show growth of spherulitic crystalline domains upon cooling after having been heated above its melting temperature. On the other hand, the complex C-[CH 2 -(OCH 2 CH 2 ) 29 -NH 3 + Cl − ] 4 ·4 I-C 10 F 21 shows a main endothermic peak at 44 °C ( Fig. 2d ) corresponding to the transition from crystalline solid to the liquid-crystalline phase (smectic A phase, SmA), as supported by POM at 47 °C, Fig. 3c . POM ( Fig. 3d ) agrees with the DSC data as the optical anisotropy is suppressed upon heating from 48 to 54 °C, and becomes again observable upon cooling. No sign of phase-separated I-C 10 F 21 or C-[CH 2 -(OCH 2 CH 2 ) 29 -NH 3 + Cl − ] 4 polymer was observed. The present finding shows the first observation of supramolecular halogen-bonded liquid crystals involving polymers. 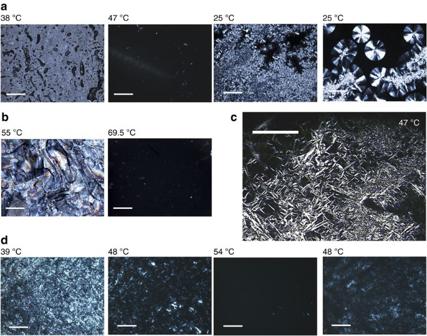Figure 3: Polarized optical micrographs. (a) C-[CH2-(OCH2CH2)29-NH3+Cl−]4after heating to 38 and 47 °C, subsequent cooling and resting at room temperature for about 5 min. The growth of crystalline spherulitic domains is observed over time upon cooling below the polymer’s melting temperature. (b) I-C10F21.(c) C-[CH2-(OCH2CH2)29-NH3+Cl−]4·4 I-C10F21complex at 47 °C, suggesting smectic A-type liquid crystallinity (SmA), as prepared by grinding. (d) C-[CH2-(OCH2CH2)29-NH3+Cl−]4·4 I-C10F21complex after heating to 39, 48 and 54 °C, and subsequent cooling to 48 °C. The complex is prepared from isopropanol solution. Scale bars, 200 μm. Figure 3: Polarized optical micrographs. ( a ) C-[CH 2 -(OCH 2 CH 2 ) 29 -NH 3 + Cl − ] 4 after heating to 38 and 47 °C, subsequent cooling and resting at room temperature for about 5 min. The growth of crystalline spherulitic domains is observed over time upon cooling below the polymer’s melting temperature. ( b ) I-C 10 F 21. ( c ) C-[CH 2 -(OCH 2 CH 2 ) 29 -NH 3 + Cl − ] 4 ·4 I-C 10 F 21 complex at 47 °C, suggesting smectic A-type liquid crystallinity (SmA), as prepared by grinding. ( d ) C-[CH 2 -(OCH 2 CH 2 ) 29 -NH 3 + Cl − ] 4 ·4 I-C 10 F 21 complex after heating to 39, 48 and 54 °C, and subsequent cooling to 48 °C. The complex is prepared from isopropanol solution. Scale bars, 200 μm. Full size image Halogen-bonded mesogen directed self-assembly The structures were elucidated by using small-angle X-ray scattering (SAXS), X-ray diffraction (XRD) and transmission electron microscopy (TEM) ( Fig. 4 ). As a reference, the pristine C-[CH 2 -(OCH 2 CH 2 ) 29 -NH 3 + Cl − ] 4 shows a nanoscale periodicity due to the charge clustering of the end-group ammonium salts, as SAXS shows a broad reflection at q 2 =0.067 Å −1 (periodicity of ca. 9.4 nm) with a faint second-order reflection ( Fig. 4a , plot 2). Two-dimensional (2D) SAXS confirms that the material is macroscopically isotropic with a poor overall alignment. Peaks q 5 and q 6 ( Fig. 4b , plot 2) are signatures of the crystalline structure within C-[CH 2 -(OCH 2 CH 2 ) 29 -NH 3 + Cl − ] 4 . Pure I-C 10 F 21 shows a reflection at q 1 =0.38 Å −1 (periodicity of ca. 1.6 nm) (see Fig. 4a , plot 1) and its higher-order peaks in the wide-angle region ( Fig. 4b , plot 1). On the other hand, the complex C-[CH 2 -(OCH 2 CH 2 ) 29 -NH 3 + Cl − ] 4 ·4 I-C 10 F 21, as prepared from isopropanol solution, shows a highly ordered lamellar structure with the primary SAXS peak at q 3 =0.055 Å −1 and a series of higher-order reflections 2 q 3 , 3 q 3 , 4 q 3 and 5 q 3 ( Fig. 4a , plot 3). Compared with the pure polymer, the periodicity has increased to 11.4 nm, due to the intercalation of the halogen-bonded I-C 10 F 21 mesogens ( Fig. 4d ). XRD shows narrow reflections at q 4 =1.4 Å −1 , 2 q 4 and 3 q 4 corresponding to a well-defined spacing of 0.45 nm ( Fig. 4b , plot 3), which suggests tight lateral packing driven by the perfluoroalkyl rod-like chains. Peak q 5 ( Fig. 4b , plot 3) indicates crystallization within the C-[CH 2 -(OCH 2 CH 2 ) 29 -NH 3 + Cl − ] 4 domains. 2D SAXS shows improved overall alignment in comparison with the pure polymer, which is also confirmed by TEM ( Fig. 4c ). As C-[CH 2 -(OCH 2 CH 2 ) 29 -NH 3 + Cl − ] 4 ·4 I-C 10 F 21 shows no SAXS reflections of the starting materials, macroscopic phase separation is not suggested. 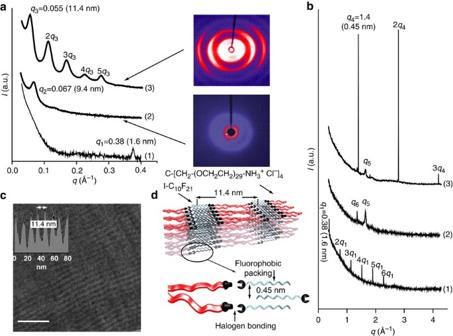Figure 4: Self-assembly due to complexation with I-C10F21. (a) SAXS patterns of I-C10F21(1), C-[CH2-(OCH2CH2)29-NH3+Cl−]4(2, indicating poor self-assembly by segregation of the ionic end-groups from the polyethylene glycol-core), and supramolecular complex C-[CH2-(OCH2CH2)29-NH3+Cl−]4·4 I-C10F21(3, showing highly ordered self-assembly). Corresponding 2D SAXS (right) shows poor overall order for C-[CH2-(OCH2CH2)29-NH3+Cl−]4and high overall order for C-[CH2-(OCH2CH2)29-NH3+Cl−]4·4 I-C10F21. (b) XRD shows (1) fluoroalkyl chain order for pure I-C10F21, (2) Polyethylene glycol-crystallization for pure C-[CH2-(OCH2CH2)29-NH3+Cl−]4and (3) lateral packing due to the fluoroalkyl chains in the supramolecular complex C-[CH2-(OCH2CH2)29-NH3+Cl−]4·4 I-C10F21. (c) TEM micrograph of C-[CH2-(OCH2CH2)29-NH3+Cl−]4·4 I-C10F21, showing lamellar smectic-like order with periodicity of 11.4 nm (scale bar, 50 nm). (d) Cartoon showing the self-assembly mechanism of the halogen-bonded complex. Figure 4: Self-assembly due to complexation with I-C 10 F 21 . ( a ) SAXS patterns of I-C 10 F 21 ( 1 ), C-[CH 2 -(OCH 2 CH 2 ) 29 -NH 3 + Cl − ] 4 ( 2 , indicating poor self-assembly by segregation of the ionic end-groups from the polyethylene glycol-core), and supramolecular complex C-[CH 2 -(OCH 2 CH 2 ) 29 -NH 3 + Cl − ] 4 ·4 I-C 10 F 21 ( 3 , showing highly ordered self-assembly). Corresponding 2D SAXS (right) shows poor overall order for C-[CH 2 -(OCH 2 CH 2 ) 29 -NH 3 + Cl − ] 4 and high overall order for C-[CH 2 -(OCH 2 CH 2 ) 29 -NH 3 + Cl − ] 4 ·4 I-C 10 F 21 . ( b ) XRD shows ( 1 ) fluoroalkyl chain order for pure I-C 10 F 21 , ( 2 ) Polyethylene glycol-crystallization for pure C-[CH 2 -(OCH 2 CH 2 ) 29 -NH 3 + Cl − ] 4 and ( 3 ) lateral packing due to the fluoroalkyl chains in the supramolecular complex C-[CH 2 -(OCH 2 CH 2 ) 29 -NH 3 + Cl − ] 4 ·4 I-C 10 F 21 . ( c ) TEM micrograph of C-[CH 2 -(OCH 2 CH 2 ) 29 -NH 3 + Cl − ] 4 ·4 I-C 10 F 21 , showing lamellar smectic-like order with periodicity of 11.4 nm (scale bar, 50 nm). ( d ) Cartoon showing the self-assembly mechanism of the halogen-bonded complex. Full size image The high order in the complex C-[CH 2 -(OCH 2 CH 2 ) 29 -NH 3 + Cl − ] 4 ·4 I-C 10 F 21 observed by X-ray scattering and TEM can be explained by the interplay between various interactions. First, I-C 10 F 21 interacts through a halogen bond with the chloride ion of the ammonium chloride end-capped polyethylene glycol polymer chains. Then, the terminal perfluoroalkyl rod-like chains pack tightly into fluorous-segregated layers, resulting in a long-range lamellar order, which can even be improved by annealing at mild conditions. Indeed, in Fig. 5 we show that vacuum treatment at sufficiently low temperature does not cause removal of I-C 10 F 21 from the complexes. For that, C-[CH 2 -(OCH 2 CH 2 ) 29 -NH 3 + Cl − ] 4 ·4 I-C 10 F 21 was kept in high vacuum for 2 days at 33 o C, which is below the melting point of the crystalline domains within the C-[CH 2 -(OCH 2 CH 2 ) 29 -NH 3 + Cl − ] 4 phase. In these conditions the complex remains stable, as seen from the C-F (1,206 cm −1 ) stretching and I-CF 2 (643 cm −1 ) deformation bands in Fig. 5a as compared with those shown in Fig. 2a . Such a vacuum annealing at low temperature even slightly improves the structural order and overall alignment of the system, compared with non-annealed sample (see Fig. 5b ), showing primary SAXS peak at q 1 =0.052 Å −1 and a series of higher-order reflections, as shown in Fig. 5b . 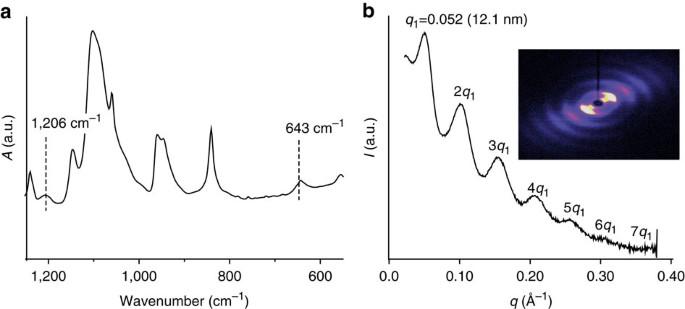Figure 5: Stability of the complex below the melting point. (a) FTIR and (b) SAXS showing structural and chemical stability of the C-[CH2-(OCH2CH2)29-NH3+Cl−]4·4 I-C10F21complex measured after high-vacuum treatment at 33 °C. Figure 5: Stability of the complex below the melting point. ( a ) FTIR and ( b ) SAXS showing structural and chemical stability of the C-[CH 2 -(OCH 2 CH 2 ) 29 -NH 3 + Cl − ] 4 ·4 I-C 10 F 21 complex measured after high-vacuum treatment at 33 °C. Full size image However, I-C 10 F 21 can be completely removed upon thermal treatment at sufficiently high temperatures, as demonstrated by the thermogram obtained in the second heating cycle ( Supplementary Fig. 2 ), which coincides with that of pure C-[CH 2 -(OCH 2 CH 2 ) 29 -NH 3 + Cl − ] 4 ( Fig. 2d ). It appears, therefore, that all of I-C 10 F 21 has been removed during the heating to 90 °C in the first cycle. It is important to note that at mild conditions, that is, vacuum and mild temperatures, the complex remains stable. We next aimed to further reduce the interfacial curvature and undulations. Therefore, we incorporated a longer fluorous tail by using I-C 12 F 25 to increase the repulsion to the organic domains. However, since 1-iodoperfluorododecane is poorly soluble in common organic solvents, we could not use solution methods to prepare the complexes. Here we identified a vapour-phase procedure as a facile and new processing method to prepare the complex by exposing drop-cast films of C-[CH 2 -(OCH 2 CH 2 ) 29 -NH 3 + Cl − ] 4 to vapours of I-C 12 F 25 at ca. 100 °C for 3 h. This allowed the volatile I-C 12 F 25 to penetrate the melt polymer and become absorbed by forming halogen bonds. The films can even be relatively thick, even a fraction of millimetre. After the reaction, the material was returned back to room temperature and analysed by XPS ( Fig. 2b,c ) and FTIR ( Supplementary Fig. 1 ; Supplementary Note 3 ), which showed occurrence of halogen bonding of I-C 12 F 25 to C-[CH 2 -(OCH 2 CH 2 ) 29 -NH 3 + Cl − ] 4 . Such longer perfluoroalkyl chains led to increased thickness of the fluorous layer, as SAXS showed the main reflection at q 2 ≈0.05 Å −1 ( Fig. 6a , plot 2), indicating that periodicity has increased from 9 nm ( Fig. 6a , plot 1) to 12.5 nm. This agrees with the halogen bond-driven intercalation of I-C 12 F 25 upon complexing with the polymer, followed by interdigitation and packing of the perfluoroalkyl chains, which result into a highly ordered and oriented lamellar structure, as demonstrated by higher-order reflections 2 q 2 , 3 q 2 and 4 q 2 ( Fig. 6a , plot 2) and 2D SAXS ( Fig. 6b ). However, the most striking observation was based on TEM. TEM micrographs on several positions provided direct evidence that there is an overall alignment of the C-[CH 2 -(OCH 2 CH 2 ) 29 -NH 3 + Cl − ] 4 ·4 I-C 12 F 25 complex, which extends to the millimetres ( Fig. 6d ), that is, six orders of magnitude higher than the nanometric-scale interactions and assembly, as driven by the halogen bonding and fluorophobic effect. The starting polymer ( Fig. 6c ) or complexes with IPFAs shorter than 10 carbon atoms do not show such an overall alignment. The I-C 12 F 25 can also be completely removed upon combined vacuum/thermal treatment, as confirmed by FTIR analysis ( Supplementary Fig. 3 ; Supplementary Note 4 ) and SAXS, which showed a shrinking of the periodicity from 12.5 nm to 9.5 nm ( Fig. 6a,b plot 3). 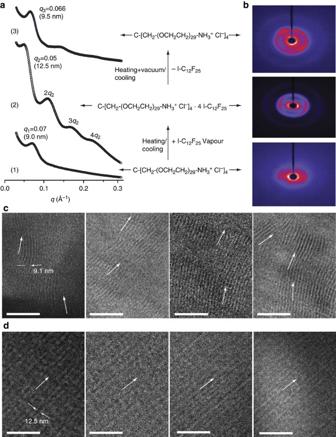Figure 6: Self-assembly due to complexation with I-C12F25. (a,b) SAXS patterns showing weak nanometer-scale order of the pristine C-[CH2-(OCH2CH2)29-NH3+Cl−]4(1); halogen bonding leads to an increased periodicity by complexation of I-C12F25from vapours at ca. 100 °C to C-[CH2-(OCH2CH2)29-NH3+Cl−]4and allows highly ordered self-assembly with equidistant reflections based on SAXS (2) and high overall alignment. By heating and vacuum treatment, the halogen-bonded I-C12F25is removed and the original periodicity is approximately recovered, however, showing better residual alignment of C-[CH2-(OCH2CH2)29-NH3+Cl−]4(3). (c) TEM micrographs at various points of pure C-[CH2-(OCH2CH2)29-NH3+Cl−]4showing lack of macroscale alignment. (d) TEM micrographs of the complex C-[CH2-(OCH2CH2)29-NH3+Cl−]4·4 I-C12F25, denoted as its nominal composition, after 3 h of exposure to I-C12F25vapours. The micrographs were taken at spots ~0.5 mm apart from each other, and show exceptionally well-ordered lamellar nanostructures with overall macroscale order at the millimetre scale. Scale bar, 100 nm (c,d). Figure 6: Self-assembly due to complexation with I-C 12 F 25 . ( a , b ) SAXS patterns showing weak nanometer-scale order of the pristine C-[CH 2 -(OCH 2 CH 2 ) 29 -NH 3 + Cl − ] 4 ( 1 ); halogen bonding leads to an increased periodicity by complexation of I-C 12 F 25 from vapours at ca. 100 °C to C-[CH 2 -(OCH 2 CH 2 ) 29 -NH 3 + Cl − ] 4 and allows highly ordered self-assembly with equidistant reflections based on SAXS ( 2 ) and high overall alignment. By heating and vacuum treatment, the halogen-bonded I-C 12 F 25 is removed and the original periodicity is approximately recovered, however, showing better residual alignment of C-[CH 2 -(OCH 2 CH 2 ) 29 -NH 3 + Cl − ] 4 ( 3 ). ( c ) TEM micrographs at various points of pure C-[CH 2 -(OCH 2 CH 2 ) 29 -NH 3 + Cl − ] 4 showing lack of macroscale alignment. ( d ) TEM micrographs of the complex C-[CH 2 -(OCH 2 CH 2 ) 29 -NH 3 + Cl − ] 4 ·4 I-C 12 F 25 , denoted as its nominal composition, after 3 h of exposure to I-C 12 F 25 vapours. The micrographs were taken at spots ~0.5 mm apart from each other, and show exceptionally well-ordered lamellar nanostructures with overall macroscale order at the millimetre scale. Scale bar, 100 nm ( c , d ). Full size image In summary, the halogen bond-driven self-assembly of a model polymer with IPFAs resulted in a very efficient spontaneous organization up to millimetre length scale without applying external aligning fields. The concept is based on the guiding effect of halogen bonding, owing to its strength and directionality, coupled with the packing of perfluoroalkyl mesogenic rods, whose extremely high repulsion from the organic polymeric phase promotes straight interfaces, and high dynamics due to their low molecular weight, which promotes plasticization and favours progress towards energy minimum. We believe that this approach is broad and not limited to the materials reported here, as many polymers possess halogen bond-accepting groups. The facile reversibility of the binding to the IPFAs opens up a plethora of new possibilities for the processing, structure control and molecular imprinting of polymeric materials, as well as for the tuning of materials properties, such as directional wetting, transport, optical, electrical and ionic properties. Materials C-[CH 2 -(OCH 2 CH 2 ) 29 -NH 3 + Cl − ] 4 with M n =5,000 g mol −1 was purchased from Jenkem Technology USA Inc. and used without additional purification. Iodoperfluorodecane (I-C 10 F 21 ) and iodoperfluorododecane (I-C 12 F 25 ) were purchased from Apollo Scientific Ltd. and used without additional purification. The solvents in this study were used as received from commercial suppliers. FTIR Attenuated total reflectance-FTIR spectra were recorded on a Nicolet Nexus FTIR spectrometre equipped with a UATR unit. The values were given in wavenumbers and were rounded to 1 cm −1 upon automatic assignment. DSC DSC analyses were performed on a Mettler Toledo DSC823e differential scanning calorimeter, using aluminium 40 μl sample pans and Mettler STARe software for calculation. The measurements were carried out from 25 to 100 °C, with a heating rate of 10 °C min −1 (the first cycle); after this, the sample was cooled down to −20 °C with a cooling rate of 10 °C min −1 and heated again to 100 °C (the second cycle), all at 10 °C min −1 . Calibration was carried out using an indium standard and an empty pan, sealed in the same way as the sample. Sample weights of about 1–4 mg were used in the measurements. POM Liquid crystal textures ( Fig. 3 ) were studied with an Olympus BX51 POM equipped with a Linkam Scientific LTS 350 heating stage and a Sony CCD-IRIS/RGB colour video camera connected to a Sony video monitor CMA-D2. POM images were also taken as a function of temperature ( Fig. 3 ) using a Leica DM4500 P polarization microscope with a Leica DFC420 digital camera. XPS XPS spectra were recorded by Surface Science Instruments SSX-100 spectrometre using monochromated Al K α X-rays and operated at 100 W. SAXS SAXS measurements were performed with a setup consisting of a Bruker Microstar microfocus X-ray source with a rotating anode ( λ =1.54 Å) and Montel optics. The beam from the X-ray source was further adjusted by four sets of four-blade slits, which resulted in an ~1 × 1-mm beam at the sample position. The scattered beam was detected with the Hi-Star 2D area detector (Bruker). For measurements, the sample to detector distance was set to 0.59 m to capture the desired length scale in the measurements. The measured 2D scattering data is azimuthally averaged to obtain one-dimensional SAXS data. XRD XRD spectra were recorded using XRD; Panalytical X’Pert PRO MPD. CuKα1 radiation (45 kV, 40 mA, with a wavelength of 0.154060, nm) was used. TEM TEM specimens were prepared by cryo-microtoming samples below −80 °C with a Leica EM UC7 ultramicrotome to 70–150 nm thick sections. During preliminary TEM measurements, it was noticed that sections introduced from room temperature to the high vacuum (~10 −6 bar) melted and formed micrometre-sized droplets when exposed under the beam. Therefore for the actual TEM investigations, the specimens were cooled down to −187 o C after sectioning and cryotransferred to the TEM device in order to keep the sections relatively intact. Preparation of the solid mixtures by grinding In a typical preparation procedure, C-[CH 2 -(OCH 2 CH 2 ) 29 -NH 3 + Cl − ] 4 (20 mg, 4 × 10 −3 mmol) and I-C 10 F 21 (10 mg, 1.6 × 10 −2 mmol or 20 mg, 3.2 × 10 −2 mmol, respectively) were ground in an agate mortar for 5 min. The mixture was allowed to stand overnight at room temperature, then ground for further 5 min and finally characterized by DSC, attenuated total reflectance-FTIR and POM. Preparation of the iodoperfluorodecane complex from solution I-C 10 F 21 allowed preparation of complexes with C-[CH 2 -(OCH 2 CH 2 ) 29 -NH 3 + Cl − ] 4 from solution, as isopropanol was found to be a common solvent for both compounds. The complexes were prepared by dissolving I-C 10 F 21 and C-[CH 2 -(OCH 2 CH 2 ) 29 -NH 3 + Cl − ] 4 in isopropanol in a final concentration of 10 mg ml −1 and stirred overnight. After stirring, the solvent was evaporated at room temperature and atmospheric pressure in a glass vial. Preparation of the complex by exposing to iodoperfluorododecane vapours No common solvent was found for I-C 12 F 25 and C-[CH 2 -(OCH 2 CH 2 ) 29 -NH 3 + Cl − ] 4. The latter compound was dissolved in isopropanol and cast on a glass substrate to form a film of sub-millimetre thickness by solvent evaporation. Alternatively, the C-[CH 2 -(OCH 2 CH 2 ) 29 -NH 3 + Cl − ] 4 solution was placed on a Teflon plate and inserted on a glass substrate or into a flask. In both cases the melted material was exposed to I-C 12 F 25 vapours at 100 °C for 3 h. After cooling to room temperature, the material was detached from the substrate, collected and characterized. No separate I-C 12 F 25 or C-[CH 2 -(OCH 2 CH 2 ) 29 -NH 3 + Cl − ] 4 XPS peaks ( Fig. 2b,c ) were detected, which suggests that the halogen-bonded complex is stoichiometric. Note that even relatively thick samples could be complexed. How to cite this article: Houbenov, N. et al. Halogen-bonded mesogens direct polymer self-assemblies over millimetre length scale. Nat. Commun. 5:4043 doi: 10.1038/ncomms5043 (2014).